Repopulation of decellularized mouse heart with human induced pluripotent stem cell-derived cardiovascular progenitor cells Heart disease is the leading cause of death in the world. Heart tissue engineering holds a great promise for future heart disease therapy by building personalized heart tissues. Here we create heart constructs by repopulating decellularized mouse hearts with human induced pluripotent stem cell-derived multipotential cardiovascular progenitor cells. We show that the seeded multipotential cardiovascular progenitor cells migrate, proliferate and differentiate in situ into cardiomyocytes, smooth muscle cells and endothelial cells to reconstruct the decellularized hearts. After 20 days of perfusion, the engineered heart tissues exhibit spontaneous contractions, generate mechanical force and are responsive to drugs. In addition, we observe that heart extracellular matrix promoted cardiomyocyte proliferation, differentiation and myofilament formation from the repopulated human multipotential cardiovascular progenitor cells. Our novel strategy to engineer personalized heart constructs could benefit the study of early heart formation or may find application in preclinical testing. In the United States, approximately one person dies every 34 s as a consequence of heart disease, and >5 million individuals suffer from heart failure, a disabling and frequently fatal disease [1] , [2] . Given the scarcity of organs for transplantation, end-stage heart failure is irreversible. Over 50% of patients with heart disease do not respond to current pharmacological therapies [2] . Thus the treatment of heart disease requires the development of novel and personalized therapeutic strategies, such as disease-specific pharmacological agents and patient-specific cardiac tissues for transplantation. Heart tissue engineering holds a great promise for those therapies based on the reconstruction of patient-specific cardiac muscle. To engineer three-dimensional (3D) heart tissues, a resource of heart cells and a 3D heart scaffold, allowing the seeded cells to attach and to grow, are two major components. A number of synthetic or natural derived matrixes have been used for engineering heart tissues [3] , [4] , [5] , [6] , [7] , [8] . However, most synthetic matrixes have a problem of biocompatibility [7] . More recently, a pioneering study by Ott et al . [9] generated bioartificial rat hearts by reseeding neonatal rat cardiomyocytes (CMs) into decellularized rat hearts. Since then, intact 3D scaffolds have been generated from various organs and species [10] , [11] , [12] , [13] . The major advantage of using decellularized whole heart over other matrixes is that the decellularized heart preserves the original 3D architecture and complex natural heart extracellular matrix (ECM). These are critical for reconstructing both the myocardium and vascular structures. However, due to the limited availability of human CMs, human heart tissue engineering has remained largely unexplored. Recent breakthroughs in induced pluripotent stem cells (iPSCs) established the feasibility of generating unlimited CMs from humans [14] , [15] , [16] . Compared with CMs directly isolated from patients under heart transplantation with end-stage heart diseases, human iPSC-derived CMs are renewable and free of prolonged pharmaceutical treatment. Thus, human iPSCs and the decellularized whole-heart ECMs (DC-ECMs) theoretically provide a novel platform for making personalized heart tissues. A previous study reported the repopulation of decellularized hearts using human undifferentiated embryonic stem (ES) cells [17] . However, contractility and electrical activity were not detected in those engineered heart tissues [17] . In this report, we engineered human heart tissues by repopulating whole decellularized mouse hearts with human iPS cell-derived multipotential cardiovascular progenitors (MCPs) [18] , [19] . The seeded MCPs differentiated in situ into CMs, smooth muscle cells (SMCs) and endothelial cells (ECs) with high efficiency, which reconstructed the decellularized mouse hearts. The recellularized DC-ECMs (RC-DC-ECMs) exhibited myocardium and vessel-like structures, contracted spontaneously with a rate of 40–50 beats per min, exhibited intracellular Ca 2+ transients (CaiT) and responded as expected to various drug interventions. In addition, we found that heart ECM could promote proliferation, specific cell differentiation and myofilament formation of CMs from the repopulated human MCPs. Therefore, this study established a novel strategy of human heart tissue engineering, which could be beneficial to study heart development, and future preclinical applications. 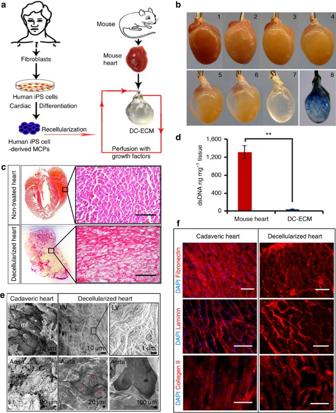Figure 1: Decellularization of mouse heart. (a) A scheme for the whole study. (b) Photographs showing each step of decellularization process: before decellularization (1); after deionized water perfusion (2); after PBS perfusion (3); after enzymatic perfusion (4); after 1% SDS solution perfusion (5); after 3% Triton X-100 solution perfusion (6); after acidic perfusion (7); perfusion of DC-ECMs with trypan blue solution to visualize the intact coronary vasculature (8). (c) H&E staining of sections from the cadaveric mouse heart (top) and DC-ECM (bottom). Scale bars, 10 μm. (d) DNA content quantification of cadaveric mouse hearts and DC-ECMs. Error bars show s.e.m of three independent experiments. **P<0.005 (n=3, unpaired Student’st-test). (e) SEM of cadaveric and decellularized hearts. Left ventricular (LV; top panel) and aorta (bottom panel). Myofibers (mf) were present in the cadaveric heart (white stars) but not in the DC-ECMs. Red stars indicate the aortic valve leaflets. (f) Immunostaining of cadaveric mouse hearts and DC-ECMs. Fibronectin (upper), Laminin (middle), and Collagen II (lower). No nuclear staining (DAPI) was observed in DC-ECMs. Scale bars, 50 μm. Mouse cadaveric heart decellularization and characterization Figure 1a illustrates the overall schema for this study. We modified a previously published decellularization protocol [10] of porcine hearts to decellularize cadaveric mouse hearts. Trypsin and detergents, including SDS and Triton X-100, were used to lyse the cellular content in mouse hearts ( Fig. 1b ). We only treated mouse hearts with peracetic acid with a low concentration for 5 min, followed with multiple washes. This process minimizes the damages on ECM proteins and properly maintains the 3D architecture of decellularized hearts, as previously described [10] . A completely decellularized heart was obtained with the yield of a transparent ECM scaffold ( Fig. 1b , panel 7). Coronary vessel tree within the DC-ECM was preserved post decellularization and was visualized with the injection of trypan blue solution through the connected cannula ( Fig. 1b , panel 8). Histological analysis by hematoxylin and eosin (H&E) staining detected no remaining nuclei in the whole decellularized hearts ( Fig. 1c ). DNA content within the decellularized hearts decreased to ~3% of that from the cadaveric mouse hearts ( Fig. 1d ). The acellular DC-ECMs were then subjected to scanning electron microscope (SEM) ( Fig. 1e ). ECM composition of the decellularized heart was preserved and exhibited a filament-like appearance ( Fig. 1e , top right panel). Aortic wall and valve leaflets remained intact in the decellularized hearts ( Fig. 1e , bottom middle and right panels). Typical ECM components such as Fibronectin, Laminin and Collagen II remained post decellularization and were detected by immunostaining ( Fig. 1f ). No DAPI-positive nuclei were observed in the decellularized hearts ( Fig. 1f ), indicating the complete removal of intact heart cells. Both ECM structure and the amount of residual DNA in the decellularized mouse hearts were similar to those reported for decellularized rat hearts [9] . Figure 1: Decellularization of mouse heart. ( a ) A scheme for the whole study. ( b ) Photographs showing each step of decellularization process: before decellularization (1); after deionized water perfusion (2); after PBS perfusion (3); after enzymatic perfusion (4); after 1% SDS solution perfusion (5); after 3% Triton X-100 solution perfusion (6); after acidic perfusion (7); perfusion of DC-ECMs with trypan blue solution to visualize the intact coronary vasculature (8). ( c ) H&E staining of sections from the cadaveric mouse heart (top) and DC-ECM (bottom). Scale bars, 10 μm. ( d ) DNA content quantification of cadaveric mouse hearts and DC-ECMs. Error bars show s.e.m of three independent experiments. ** P <0.005 ( n =3, unpaired Student’s t -test). ( e ) SEM of cadaveric and decellularized hearts. Left ventricular (LV; top panel) and aorta (bottom panel). Myofibers (mf) were present in the cadaveric heart (white stars) but not in the DC-ECMs. Red stars indicate the aortic valve leaflets. ( f ) Immunostaining of cadaveric mouse hearts and DC-ECMs. Fibronectin (upper), Laminin (middle), and Collagen II (lower). No nuclear staining (DAPI) was observed in DC-ECMs. Scale bars, 50 μm. 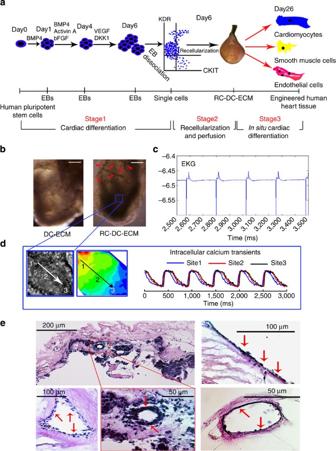Figure 2: Recellularization of decellularized mouse heart. (a) A scheme showing the working strategy to recellularize the decellularized mouse hearts with human iPSC-derived MCPs. Human iPSC-derived EBs were differentiated until day 6 and then dissociated into single cells (Stage 1). Dissociated cells (10 million) were seeded into a decellularized mouse heart and perfused (Stage 2). The seeded MCPsin situdifferentiated into cardiac lineage cells and reconstructed DC-ECMs. (b) Detection of vessel-like structures from human Y1 iPS cell recellularized DC-ECMs. Red arrows indicate the reconstructed vessel-like structures. Scale bars, 500 μm. (c) EKG recording of human Y1 iPS cell recellularized DC-ECMs when electrically paced at 4 HZ. (d) Detection of the intracellular (CaiT) synchronization driven by local propagation of electrical activity (sites 1, 2 and 3) from Y1 iPSC RC-DC-ECMs. (e) A RC-DC-ECM was embedded in paraffin and cross-sectioned, followed with H&E staining. The up left panel shows the recellularized VW. High magnification panel and the other three panels show recellularized vessel cavities and distribution of MCP-derived cells along the endocardial surface (red arrows). Full size image Differentiation of MCPs from human iPSCs Figure 2a outlines the overall workflow used to repopulate the decellularized mouse hearts with human iPSCs. At stage 1, we adapted our serum-free protocol [18] to induce the differentiation of MCPs from human Y1-iPSCs [19] ( Supplementary Fig. S1a,b ). This protocol utilizes the known role of different growth factors in early cardiovascular development to manipulate the differentiation of human ES/iPS cells to MCPs, as well as the specification of MCPs to cardiovascular lineage cells, including CMs, SMCs and ECs ( Supplementary Fig. S1c and Supplementary Movie 1 ). Embryoid bodies (EBs) were generated from Y1 iPSCs with addition of bone morphogenetic protein 4 (BMP4, 1 ng ml −1 ) for 24 h (day 0–1), followed by treatment with BMP4 (10 ng ml −1 ), basic fibroblast growth factor (bFGF, 5 ng ml −1 ) and ActivinA (1.5 ng ml −1 ) from days 1–4. Vascular endothelial growth factor A (VEGF, 10 ng ml −1 ) and dickkopf homologue 1 (DKK1, 150 ng ml −1 ) were then added from day 4 till day 6 ( Fig. 2a ). At stage 2, the day 6 EBs were dissociated into single cells. Fluorescence-activated cell sorting (FACS) analysis detected an average of 63% KDR low /C-KIT neg cells, which represented the human iPSC-derived MCPs [19] , from the dissociated EBs ( Supplementary Fig. S1d ). When further differentiated as monolayers in six-well plates, the dissociated EBs generated >50% CMs, 30% SMCs and 5% ECs with the presence of VEGF (10 ng ml −1 ) and DKK1 (150 ng ml −1 ) ( Supplementary Movie 2 ), or >10% CMs, 50% SMCs, 25% ECs in the presence of VEGF (20 ng ml −1 ) and bFGF (20 ng ml −1 ) ( Supplementary Fig. S1e ). These results indicated that cardiovascular lineage specification from iPS-MCPs could be controlled by exogenous growth factors as previously described with human ES cells [18] . Similar to our previous studies [19] , smooth muscle actin (SMA) is expressed in SMCs and CMs. Thus, the SMA+ population in Supplementary Fig. S1e represented both iPSC-derived CMs and SMCs. At Stage 3, we perfused the MCP-repopulated mouse decellularized hearts with VEGF (10 ng ml −1 ) and DKK1 (150 ng ml −1 ) to increase the reconstruction of heart muscles, or with VEGF (20 ng ml −1 ) and bFGF (20 ng ml −1 ) to promote re-endothelialization of the heart constructs. Figure 2: Recellularization of decellularized mouse heart. ( a ) A scheme showing the working strategy to recellularize the decellularized mouse hearts with human iPSC-derived MCPs. Human iPSC-derived EBs were differentiated until day 6 and then dissociated into single cells (Stage 1). Dissociated cells (10 million) were seeded into a decellularized mouse heart and perfused (Stage 2). The seeded MCPs in situ differentiated into cardiac lineage cells and reconstructed DC-ECMs. ( b ) Detection of vessel-like structures from human Y1 iPS cell recellularized DC-ECMs. Red arrows indicate the reconstructed vessel-like structures. Scale bars, 500 μm. ( c ) EKG recording of human Y1 iPS cell recellularized DC-ECMs when electrically paced at 4 HZ. ( d ) Detection of the intracellular (CaiT) synchronization driven by local propagation of electrical activity (sites 1, 2 and 3) from Y1 iPSC RC-DC-ECMs. ( e ) A RC-DC-ECM was embedded in paraffin and cross-sectioned, followed with H&E staining. The up left panel shows the recellularized VW. High magnification panel and the other three panels show recellularized vessel cavities and distribution of MCP-derived cells along the endocardial surface (red arrows). Full size image Recellularization of decellularized mouse hearts Approximately 1.0 × 10 7 of day 6 EB-dissociated single cells were seeded into one decellularized mouse heart ( Supplementary Fig. S2a ) through the cannula that was connected to the aorta. In order to induce CM formation from the seeded MCPs, heart constructs were periodically (once per 8 h) perfused with VEGF (10 ng ml −1 ) and DKK1 (150 ng ml −1 ) through the same cannula. To calculate the retention ratio of repopulated cells, we collected the perfusate and counted the total cell loss of each perfusion. After 7 days, only a few cells were observed in the medium post perfusion, suggesting a stable interaction of repopulated cells with the heart ECM had occurred. Thus, we estimated ~10–15% repopulated cells were preserved in the DC-ECMs after 7 days perfusion. In addition to Y1 iPSC-derived MCPs, we also repopulated the decellularized mouse hearts with human RUES2 ES cell-derived MCPs ( Supplementary Fig. S2b,c ). We observed reconstructed vessel-like structures within both human iPS cell and ES cell recellularized heart constructs ( Fig. 2b , Supplementary Fig. S3a ). Both ES- and iPS cell-repopulated heart constructs exhibited spontaneous contractions after 20 days of perfusion ( Supplementary Movies 3 and 4 ), with a similar beating rate of 40–50 beats per min. This observation indicated an identical cardiovascular commitment process from the repopulated MCPs of human ES cells and iPS cells. Electrophysiological analysis of engineered heart constructs Of all the constructs engineered in this study, ~90% exhibited spontaneous contractions and 10% failed to beat because of the low cell retention or contamination during perfusion. In order to examine the electrophysiological characteristics of engineered heart tissues, we first conducted EKG (electrocardiogram) recording ( Fig. 2c ). In humans, EKG is used to measure the electrical activity of whole heart and diagnose abnormal rhythms of the heart. The engineered heart constructs showed EKG-like electrical signals with irregular wave morphology, indicating the lack of electrical activities controlled by a conduction system. Next, we investigated whether CMs within the engineered heart tissues were electrically coupled by loading the RC-DC-ECMs with an intracellular Ca 2+ indicator dye, Rhod-2/AM and mapping CaiT at the high spatial and temporal resolution [20] . Figure 2d and Supplementary Fig. S3 show the optical recording of CaiT in the heart constructs engineered with human Y1 iPS and RUES2 ES cells. Mapping CaiT in a paced preparation is an outstanding surrogate for mapping action potential propagation and to measure local cell–cell coupling, as previously demonstrated [19] , [20] . CaiT mapping detected many regions of uniform wave propagation indicating a possible electrical coupling of CMs and cell–cell communication in heart constructs recellularized with pluripotent stem cells ( Fig. 2d , Supplementary Fig. S3b and Supplementary Movie 5 ). However, CaiT waves also encountered zones of anatomical block indicating regions of uncoupled tissues. The loss of coupling was most likely due to gaps between the recellularized CMs or a low density of CMs, as those uncoupled areas could be re-synchronized by electrical stimulation ( Supplementary Fig. S3b , Supplementary Movie 6 ). Optical mapping results indicated that our engineered heart constructs largely functioned as a syncytium, often with an endogenous pacemaker and otherwise could be electrically paced. Histological analysis of engineered heart constructs After 20 days of perfusion, expression of pluripotency marker genes, including NANOG , SOX2 and OCT4 , was significantly decreased in heart constructs compared with that in undifferentiated iPS cells, indicating no remaining of pluripotent iPS cells ( Supplementary Fig. S2d ). Histological analysis of engineered heart constructs revealed MCP-derived cells (detected by H&E) that formed muscle-like or vessel cavities-like structures, as well as a single layer on the endocardial surface ( Fig. 2e ). To identify the types of cells locating on the different sites of DC-ECMs, sections were immunostained using antibodies recognizing human CMs, SMCs and ECs ( Fig. 3a–c ). Myofibers were detected in the recellularized ventricular wall (VW) ( Fig. 3a ), as illustrated with low-magnification images to visualize as large a field-of-view as possible. Two CM markers, sarcomeric α-Actinin and Cardiac Troponin T (CTNT) [18] were found throughout the DC-ECMs post recellularization ( Fig. 3a ). SMA immunostaining illustrated the recellularized VW, apex (AP) and ventricular septum (VS) ( Supplementary Fig. S4a ). Both SMCs and CMs repopulated the VS and exhibited the branching structures. Immunostaining of smooth muscle myosin heavy chain (SMMHC), a marker of SMC, detected the differentiation and localization of SMCs on the border of CM fibres ( Fig. 3b ), as well as in some small vessel cavities (data not shown). ECs distribution was observed along the endocardial surface with the formation of a single layer of ECs ( Fig. 3c ). Both PECAM (CD31) and VE-Cadherin [18] expressions were detected on ECs located on the inner surface of the small coronary vessels throughout the engineered heart tissues ( Supplementary Fig. S4b ). The MCP-derived CMs refilled the decellularized mouse hearts ( Fig. 3d ) and expressed Connexin-43 (CX43), which is the predominant cardiac gap-junction protein ( Fig. 3e ). The CX43 expression pattern in our heart tissue is not as homogenous as that in native myocardium and comparable to that in previous bioartificial rat hearts [9] . Lastly, we quantified the ratios of CMs and ECs in the heart constructs after perfusion with media containing DKK1 (150 ng ml −1 ) and VEGF (10 ng ml −1 ) or VEGF (20 ng ml −1 ) and bFGF (20 ng ml −1 ). We found the presence of bFGF and DKK1 could substantially promote the specification of ECs or CMs from the reseeded human MCPs, respectively ( Fig. 3f ). These data indicated that the local heart ECM niches, as well as the extracellular growth factors, could affect the migration and/or lineage commitment of early-stage heart progenitor cells. 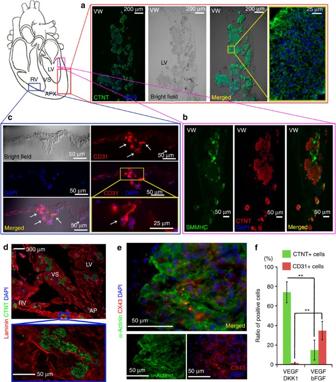Figure 3: Histology analyses of engineered heart tissues. (a) A representative coronal section of recellularized mouse heart immunostained by CTNT and merged with the bright field image. High magnification shows the sarcomeric organization of myofibers. (b) A representative VW section was immunostained with CTNT and SMMHC, a SMC marker. (c) Sections of a recellularized heart were stained by CD31, a surface mark of ECs. White arrows indicate human MCP-derived ECs along endocardial surface. (d) A representative coronal section of the recellularized mouse heart immunostained by anti-CTNT and anti- Laminin antibodies. (e) Co-immunostaining of CM marker α-Actinin and Connexin-43 (CX43), showing expression of gap-junction-associated protein in RC-DC-ECMs. Ventricular wall (VW), left ventricle (LV), right ventricle (RV), ventricle septum (VS), apex (AP). (f) Ratios of CTNT+ and CD31+ cells in the Y1 iPSC RC-DC-ECMs after perfusion with medium containing DKK1 (150 ng ml−1) and VEGF (10 ng ml−1) or VEGF (20 ng ml−1) and bFGF (20 ng ml−1). The ratio of CD31+ or CTNT+ cells in all DAPI+ cells was obtained from at least five views per section. At least 15 sections per construct were calculated. Error bars show s.e.m of three independent experiments. **P<0.01 (unpaired Student’st-test). Figure 3: Histology analyses of engineered heart tissues. ( a ) A representative coronal section of recellularized mouse heart immunostained by CTNT and merged with the bright field image. High magnification shows the sarcomeric organization of myofibers. ( b ) A representative VW section was immunostained with CTNT and SMMHC, a SMC marker. ( c ) Sections of a recellularized heart were stained by CD31, a surface mark of ECs. White arrows indicate human MCP-derived ECs along endocardial surface. ( d ) A representative coronal section of the recellularized mouse heart immunostained by anti-CTNT and anti- Laminin antibodies. ( e ) Co-immunostaining of CM marker α-Actinin and Connexin-43 (CX43), showing expression of gap-junction-associated protein in RC-DC-ECMs. Ventricular wall (VW), left ventricle (LV), right ventricle (RV), ventricle septum (VS), apex (AP). ( f ) Ratios of CTNT+ and CD31+ cells in the Y1 iPSC RC-DC-ECMs after perfusion with medium containing DKK1 (150 ng ml −1 ) and VEGF (10 ng ml −1 ) or VEGF (20 ng ml −1 ) and bFGF (20 ng ml −1 ). The ratio of CD31+ or CTNT+ cells in all DAPI+ cells was obtained from at least five views per section. At least 15 sections per construct were calculated. Error bars show s.e.m of three independent experiments. ** P <0.01 (unpaired Student’s t -test). Full size image Impact of heart ECM on CM commitment from human MCPs Previous studies demonstrated that ECM influences vertebrate heart formation [21] , [22] . It would be interesting to know the role of heart ECM in regulating early-stage human cardiovascular differentiation, and our engineered heart constructs provide an ideal model to address these questions. First, we conducted q-PCR to compare the relative expression levels of several cardiac-specific genes in undifferentiated Y1-iPSCs, day 26 Y1 EBs, day 26 heart ECM constructs, human fetal heart and human heart atrium ( Fig. 4a ). Twenty million day 6 EB cells were generated from Y1 iPS cells, of which 10 million EB cells were used to make a heart construct and the other half were cultured in six-well plates. Both EBs and heart constructs were cultured with the same medium till day 26. This allowed us to compare the CM differentiation from MCPs under two 3D environments. One 3D environment is the decellularized mouse heart ECM, whereas the other represents 3D EBs in the absence of mouse heart ECM. Expression levels of α -MHC , CTNT , CX43 and NK2 homeobox 5 ( NKX2.5 ) in heart ECMs were identical to those from the two human heart tissues and were significantly higher than those from the EBs ( Fig. 4a ). The expression level of β -MHC in heart ECMs was five-fold higher than that in the day 26 EBs. Next, we compared the expression levels of atrial CM markers, Myosin regulatory light chain 2, atrial isoform ( MLC2A ), Sarcolipin ( SLN ) [23] and ventricular CM marker, Iroquois homeobox 4 ( IRX4 ) [24] in all samples. As expected, the highest expression level of atrial markers and the lowest level of IRX4 were detected in human atrium. Interestingly, we found an increased level of IRX4 in heart ECMs than that in EBs. The relative expression ratio of IRX4 versus SLN in the heart ECMs was comparable to that in fetal heart, but significantly higher than those in EBs and human atrium ( Fig. 4b ). Additionally, a higher ratio of MLC2A+CMs was observed in the recellularized atria than in the ventricles (38 versus 17%, Fig. 4c ). However, the atria of engineered heart constructs were not recellularized as well as the ventricles, which was confirmed by both histological and q-PCR analyses ( Supplementary Fig. S5 ). Therefore, all these results implied a potential role of ventricular heart ECM during the commitment of ventricular CMs from MCPs. 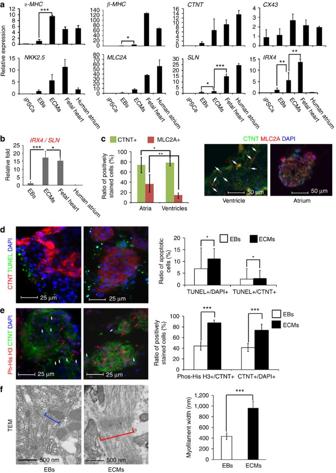Figure 4: Impact of heart ECM on repopulated MCPs. (a) Transcriptional expression of cardiac-associated genes, including cardiac-specific genes (α-MHC, β-MHC,CTNT,MLC2A,SLNandIRX4), cardiac-related transcription factor (NKX2.5), and gap-junction protein (CX43) (n=3). (b) Relative expression ratio ofIRX4versusSLNwas compared (n=3). (c) Quantification of CTNT+ and MLC2A+ cells in the recellularized atria and ventricles. Both atria and ventricles were separated from the heart constructs and subjected to MLC2A (red) and CTNT (green) immunostaining. At least 10 sections of each tissue were calculated. White arrows indicate the MLC2A+ cells in ventricles. (d) Cell apoptosis assessment. EBs and RC-DC-ECMs were stained with anti-CTNT antibody and labelled with TUNEL assay. Quantitative apoptotic nuclei in total DAPI+ or in CMs were calculated and were shown in histogram (right) (n=3). (e) Cell proliferation assessment. EBs and RC-DC-ECMs were stained with anti-CTNT and anti-phospho-Histone H3 antibodies. Quantitative proliferating nuclei in CMs and ratio of CTNT in total DAPI+ cells were calculated and shown in histogram (right) (n=3). Red arrows indicate the proliferating nuclei and white arrows indicate the phospho-Histone H3-negative nuclei. (f) Ultrastructural analysis of CMs in EBs and RC-DC-ECMs by TEM. Width of myofibrillar bundles was measured (right). F, myofibrillar bundle. Z, Z-line. All error bars show s.e.m of three independent experiments. *P>0.05, **P<0.05, ***P<0.01 (unpaired Student’st-test). Figure 4: Impact of heart ECM on repopulated MCPs. ( a ) Transcriptional expression of cardiac-associated genes, including cardiac-specific genes (α -MHC , β -MHC , CTNT , MLC2A , SLN and IRX4 ), cardiac-related transcription factor ( NKX2.5 ), and gap-junction protein ( CX43 ) ( n =3). ( b ) Relative expression ratio of IRX4 versus SLN was compared ( n =3). ( c ) Quantification of CTNT+ and MLC2A+ cells in the recellularized atria and ventricles. Both atria and ventricles were separated from the heart constructs and subjected to MLC2A (red) and CTNT (green) immunostaining. At least 10 sections of each tissue were calculated. White arrows indicate the MLC2A+ cells in ventricles. ( d ) Cell apoptosis assessment. EBs and RC-DC-ECMs were stained with anti-CTNT antibody and labelled with TUNEL assay. Quantitative apoptotic nuclei in total DAPI+ or in CMs were calculated and were shown in histogram (right) ( n =3). ( e ) Cell proliferation assessment. EBs and RC-DC-ECMs were stained with anti-CTNT and anti-phospho-Histone H3 antibodies. Quantitative proliferating nuclei in CMs and ratio of CTNT in total DAPI+ cells were calculated and shown in histogram (right) ( n =3). Red arrows indicate the proliferating nuclei and white arrows indicate the phospho-Histone H3-negative nuclei. ( f ) Ultrastructural analysis of CMs in EBs and RC-DC-ECMs by TEM. Width of myofibrillar bundles was measured (right). F, myofibrillar bundle. Z, Z-line. All error bars show s.e.m of three independent experiments. * P >0.05, ** P <0.05, *** P <0.01 (unpaired Student’s t -test). Full size image In order to study the impact of heart ECM on MCP-derived CMs, the ratios of CMs in day 26 EBs versus day 26 heart constructs were compared. Approximately 40% CMs were identified in EBs and ~70% CMs were found in heart constructs ( Fig. 4e , right). This suggested that heart ECM may have an impact on the viability of CMs. Next, we assessed the levels of cell apoptosis and proliferation. Approximately 6 and 10% apoptotic cells were detected from all DAPI+ cells within EBs and RC-DC-ECMs, respectively. Nearly 2.5% apoptotic CMs were identified in both EBs and RC-DC-ECMs ( Fig. 4d , Supplementary Fig. S6 ). Given the higher cell density and the lower delivery of nutrition supply in the heart constructs, more apoptotic cells were expected in RC-DC-ECMs than in EBs. Interestingly, we found ~80% of phospho-Histone H3-positive CMs in RC-DC-ECMs and only 40% of phospho-Histone H3 positive CMs in EBs ( Supplementary Fig. S7 , Fig. 4e ). Taken together, our results suggested that heart ECM could stimulate the proliferation of early differentiated CMs or maintain the proliferation of CMs for a longer period of time than in a 3D environment devoid of ECM. The ultrastructures of CMs in EBs and RC-DC-ECMs were investigated by TEM. We found wider myofilament bands within RC-DC-ECMs than those from the EBs ( Fig. 4f ), indicating that heart ECM may promote the formation of myofibrillar bundles in CMs. Drug response of engineered heart constructs As our engineered heart constructs exhibited spontaneous contractions, we next sought to test whether these constructs could respond to pharmaceutical agents, which are known to affect CM physiology. In clinical and experimental settings, the increase of heart beating rate in response to β-adrenergic stimulation has been well documented [25] . The chronotropic response of our heart constructs to β-adrenergic stimulation was examined by perfusing isoproterenol, a selective β1-adrenergic agonist, with concentrations ranging from 1 nM to 5 μM. As shown in Fig. 5a , isoproterenol administration increased the frequency of spontaneous contractions. Perfusion with 1 μM isoproterenol doubled the contraction rate from ~45 beats per min to 90 beats per min, and induced small premature calcium waves that gradually developing to full Ca 2+ transients ( Fig. 5b ). Next, we tested the response of RC-DC-ECMs to E4031, a selective blocker of the rapid component of the delayed rectifying K + current, I Kr , known to elicit long QT type 2 and Torsade de Pointes, a form of polymorphic ventricular arrhythmias [26] . Inhibition of I Kr with E4031 gradually developed Ca 2+ instabilities ( Fig. 5c ), resulting in an arrhythmogenic phenotype with irregular amplitude of Ca 2+ transient ( Fig. 5d ) compared with the baseline conditions. This observation is consistent with the report that Ca 2+ instability or lability often precedes ventricular arrhythmias in drug-induced long QT type 2 (ref. 27 ). Furthermore, we measured the baseline mechanical force, as well as the active force of heart constructs in response to external [Ca 2+ ] out , as previously described [28] . Supplementary Fig. S8 shows a representative image of a heart construct instrumented to measure mechanical force. Engineered heart tissues generated contractile force by spontaneous contractions and showed increased contractile force in response to increased [Ca 2+ ] out ( Fig. 5e,f , Supplementary Movie 7 ). Active force–frequency relationship showed that active contractile force was increased with electrical pacing between 1 to 1.5 Hz and then decreased at 2 and 2.5 Hz ( Fig. 5g , Supplementary Movie 8 ), which is consistent with the stair-case effect observed in the working myocardium [29] . The average contraction force of engineered heart constructs under 1-Hz pacing was ~0.18 mN, which was higher than the force generated by spontaneous contractions and comparable to another report on engineered human heart tissues [30] . Put together, these results indicated that the heart tissues engineered with our strategy displayed electrophysiological and mechanical properties. 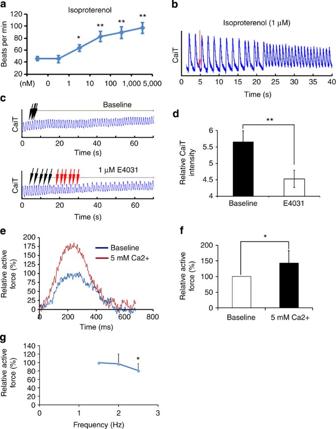Figure 5: Drug response and mechanical testing of engineered heart constructs. (a) Contraction rate recording of RC-DC-ECMs in response to isoproterenol treatment. Error bars show s.e.m of five independent experiments. *P<0.05; **P<0.01. (one-factor repeated ANOVA withpost hoctest). (b) Increased automaticity of RC-DC-ECMs in response to 1 μM isoproterenol. Red arrow indicates the time point of isoproterenol administration. (c) Inhibition ofIKrwith E4031 resulted in CaiT alternans (red arrows) and decreased CaiT intensity (d) (n=3. **P<0.01). (e) Representative active force tracing of electrically stimulated RC-DC-ECMs at 1.5 Hz. The active contractile force was increased in response to 5 mM extracellular Ca2+concentration. Blue colour indicates the tracing of baseline active force (1.25 mM Ca2+) and red-colour tracing is with 5 mM Ca2+. (f) Statistical analysis of force change in response to increase of extracellular Ca2+. (n=3. *P<0.05). (g) Change of active force in response to electrical stimulations. (n=3. 2.5 Hz versus 1.5 Hz. *P<0.05.) All error bars, except those in panela, show s.e.m of three independent experiments (unpaired Student’st-test). Figure 5: Drug response and mechanical testing of engineered heart constructs. ( a ) Contraction rate recording of RC-DC-ECMs in response to isoproterenol treatment. Error bars show s.e.m of five independent experiments. * P <0.05; ** P <0.01. (one-factor repeated ANOVA with post hoc test). ( b ) Increased automaticity of RC-DC-ECMs in response to 1 μM isoproterenol. Red arrow indicates the time point of isoproterenol administration. ( c ) Inhibition of I Kr with E4031 resulted in CaiT alternans (red arrows) and decreased CaiT intensity ( d ) ( n =3. ** P <0.01). ( e ) Representative active force tracing of electrically stimulated RC-DC-ECMs at 1.5 Hz. The active contractile force was increased in response to 5 mM extracellular Ca 2+ concentration. Blue colour indicates the tracing of baseline active force (1.25 mM Ca 2+ ) and red-colour tracing is with 5 mM Ca 2+ . ( f ) Statistical analysis of force change in response to increase of extracellular Ca 2+ . ( n =3. * P <0.05). ( g ) Change of active force in response to electrical stimulations. ( n =3. 2.5 Hz versus 1.5 Hz. * P <0.05.) All error bars, except those in panel a , show s.e.m of three independent experiments (unpaired Student’s t -test). Full size image The classic heart tissue engineering approach is to mix beating CM, together with other cardiac cells, into biomaterials to generate a layer of beating cardiac tissue. Most heart tissues were engineered with neonatal CMs from rodents [7] . In addition, most scaffolds have no preserved 3D architectures to support the rebuilding of muscle and vascular structures. Decellularized whole hearts preserve the natural matrix components and local niches, providing intact heart scaffolds needed to engineer 3D heart tissues or bioartificial hearts. Previous attempts at repopulating decellularized mouse hearts with undifferentiated human ES cells failed to generate functional heart constructs because of the low CM differentiation efficiency [17] . In this study, we succeeded in engineering functional human heart tissues by repopulating intact decellularized mouse hearts with human iPS cell-derived MCPs. MCPs represent the earliest heart progenitors in human heart development. Here we delivered MCPs through coronary vessels and took advantage of the spontaneous migration, differentiation and proliferation of MCPs in the decellularized hearts. This study for the first time utilizes human cardiovascular progenitor cells for heart tissue engineering. Moreover, by adding different growth factors in the perfusion medium, we could control the progress of re-endothelialization or of the muscle formation in the decellularized hearts. Although human heart tissues were engineered using whole mouse-heart scaffolds, we do not think that they are similar to the previously reported bioartificial rat hearts [9] . The mechanical force generated by our engineered heart tissues was insufficient for pumping blood and the whole engineered constructs were not fully synchronized. Compared to native human heart, the slow electric conduction and abnormal electrograms in our engineered heart constructs may be caused by the lack of gap-junctions, limited number of CMs, as well as the lack of a cardiac conduction system. Additionally, we didn’t observe substantial numbers of fibroblasts in heart tissues (data not shown), which was consistent with our previous finding that fibroblasts were not differentiated from MCPs [18] , [19] . Cardiac fibroblasts have an important role in regulating heart functions, including electrical conduction, and respond to myocardial contractions [31] . Therefore, it would be interesting to test whether the co-repopulation of DC-ECMs with cardiac fibroblasts and MCPs might improve the synchronization of whole engineered heart constructs. Altogether, a major challenge of this study is how to improve the electrical propagation and mechanical force of heart constructs. Our engineered heart tissues generated mechanical forces and exhibited the expected electrophysiological characteristics and normal responses to various pharmaceutical agents. All these indicated the potential preclinical applications of our engineered heart tissues. In addition, our platform for heart tissue engineering could provide an in vitro system to study the early events of human heart development. For example, it could be used to study whether and how heart ECM has an impact on early human CM differentiation, proliferation and maturation from heart progenitors. We observed appropriate cell composites in engineered tissues as seen in native heart, where CMs reconstructed the VWs and septum, and ECs formed the monolayer lining the internal surface of vessel cavity and endocardium. Thus, this system could be used to study whether different niches within cardiac ECM could regulate the lineage specification of MCPs, or the migration of MCP-derived heart cells. In general, the method used to engineer heart tissue involves the mixing of functional cardiac cells with bio-matrices. Our strategy differs in that it takes advantage of the whole-heart ECM and human early-stage heart progenitors to rebuild functional heart tissues and ultimately incorporates tissue engineering, stem cell biology and heart developmental biology into a new platform for both basic and preclinical applications. As the non-synchronized heart tissue may form an arrhythmogenic substrate, our ongoing studies are focused on improving the mechanical force and electrical synchronization and on making heart tissues from iPS cells of patients with inherited heart diseases. Perfusion decellularization of mouse hearts We used 12–16-week-old C57BL6/J mice in this study. All experimental procedures and protocols involving mice were approved by the Institutional Animal Care and Use Committee and conformed to US Animal Welfare Act and institutional guidelines. Briefly, mice were killed and the ascending aorta was cannulated with a blunted 20-gauge needle that was sutured to allow retrograde coronary perfusion. The cannulated heart was removed from the chest and kept frozen at −80 °C. Before decellularization, hearts were thawed at room temperature for 30 min and connected to a perfusion pump (Masterflex L/S Drive EW-07553-80; Cole-Parmer, Vernon Hills, Illinois, USA). Hearts were perfused with deionized water for 10 min at 1.5 ml min −1 , twice with phosphate-buffered saline (PBS) (10 min each time), 0.02% trypsin/0.05% ethylenediaminetetraacetic acid (EDTA)/0.05% NaN3 solution for 20 min, 1% sodium dodecyl sulphate (SDS)/0.05% NaN3 solution for 10 min, 3% Triton X-100/0.05% EDTA/0.05% NaN3 for 10 min, followed by a 4% deoxycholic acid solution for 5–10 min at room temperature. Disinfection was carried out by perfusion of 0.1% peracetic acid/4% ethanol for 10 min. The acid was neutralized and removed by perfusing with PBS (pH 7.4) and deionized water two times for 15 min. Decellularized hearts were immediately used or stored in PBS at 4 °C for further applications. Histology and immunofluorescence Mouse cadaveric hearts and decellularized hearts were paraffin-embedded and sectioned, followed with H&E staining. In addition, both mouse cadaveric hearts and decellularized ECMs were subjected to cryosection and immunostained with antibodies against Fibronectin (Thermo Fisher Scientific, Fremont, California, USA), Laminin (Thermo Fisher Scientific), and Collagen II (Thermo Fisher Scientific). The recellularized heart tissues were subjected to cryosection and immunostained with the following antibodies at a 1:200 dilution ratio: anti-human PECAM1 (CD31) and anti-human VE-Cadherin (R&D System); anti-human Troponin T (CTNT) and anti-human SMA (Lab Vision); anti-human-Connexin-43 (Chemicon); anti-human α-Actinin (Sigma); anti-SMMHC (DakoCytomation). All secondary antibodies were from Invitrogen. Images were recorded with OpenLab 5.5.1 (Improvisation) on a Leica DMRA microscope (Leica). The ratios of positively stained cells were quantified by counting the ratios of positively labelled cells in DAPI+ cells or CTNT+ cells. At least 10 sections per tissue and three engineered tissues were calculated. DNA quantification Approximately 25 mg of cadaveric heart ( n =3) and DC-ECM ( n =3) each were subjected to DNA extraction using DNeasy Blood & Tissue kit (QIAGEN, Valencia, California, USA) according to the manufacturer’s instructions. The DNA extracts were next used for DNA quantification. A Quant-iT PicoGreen dsDNA Assay kit (Invitrogen) was used to measure the amount of DNA. The fluorescence reading (excitation 485 nm and emission 528 nm) was taken on a microplate reader, and the absolute amount of DNA (ng ml −1 ) was quantified against a lambda DNA standard curve (0 ng ml −1 –1 μg ml −1 ). Scanning electron microscopy (SEM) DC-ECMs and cadaveric hearts were fixed with 2.5% (vol/vol) glutaraldehyde for 1 h at room temperature, followed by washing with PBS for three times (15 min each) and post-fixed with 1% osmium tetroxide for 1 h. After osmium tetroxide fixation, the tissue was extensively washed in PBS, followed with serial dehydration using 30, 50, 70, 90 and 100% ethanol and hexamethyldisilazane, and then air-dried. Samples were coated with 3.5-μm AuPd using a Cressington sputter coater system (sputter module 108auto, Cressington Scientific, Watford, UK). Standard scanning electron digitized images were captured with a Jeol 6335F field emission SEM with backscatter detector (Jeol, Tokyo, Japan). Transmission electron microscopy (TEM) EBs and RC-DC-ECMs were fixed using 2.5% glutaraldehyde in 0.1 M PBS (pH 7.4) for 10 min, followed with three washes with PBS (15 min each) and post-fixed with 1% osmium tetroxide containing 1% potassium ferricyanide for 1 h. The fixed samples were washed in PBS, dehydrated in an ethanol series: 30, 50, 70, 90 and 100% for 15 min each time and then in propylene oxide for 10 min. Next samples were infiltrated with epon by a propylene oxide/epon series starting with 1:1 for 3 h, then three times in 100% epon (1 h each time). The samples were then embedded in moulds containing 100% epon and polymerized at 60 °C overnight, followed with being sectioned at about 80-nm thickness and stained with lead citrate for 8 min. Electron micrographs were taken using a JEOL JEM-1011 transmission electron microscope (JEOL, Germany). Cell culture and differentiation The human Y1 iPSCs [19] and human RUES2 ES cells (Rockefeller University) were maintained on mitotically inactivated MEFs in human ES cell medium containing DMEM/F12 (Invitrogen), 20% (vol/vol) KSR (Invitrogen), 1% penicillin/streptomycin (Invitrogen), 2 mM L-glutamine (Invitrogen), 0.1 mM non-essential amino acids (Invitrogen), 0.05 mM β-mercaptoethanol (β-ME, Sigma-Aldrich, St Louis, Missouri, USA) and 10 ng ml −1 bFGF. The following conditions were used for cardiovascular differentiation using the basal StemPro-34 (invitrogen) medium: day 0–1, BMP4 (1 ng ml −1 ); day1–4, BMP4 (20 ng ml −1 ), bFGF (5 ng ml −1 ) and ActivinA (3 ng ml −1 ); day4–8, DKK1 (150 ng ml −1 ) and VEGF (10 ng ml −1 ); after day 8, VEGF (10 ng ml −1 ) and DKK1 (150 ng ml −1 ). Cultures were maintained in a 5% CO 2 /5% O 2 environment. All cytokines were from R&D Systems. Recellularization of decellularized mouse hearts DC-ECMs were washed using water (Cellgro, Manassas, Virginia, USA), PBS (Invitrogen) and DMEM (Invitrogen) for 30 min each. Day 6 EBs were harvested, dissociated to single cells with trypsin (0.25% trypsin-EDTA). Approximately 1.0 × 10 7 cells were suspended in basic differentiation media (StemPro-34, Invitrogen) containing 2 mM glutamine, 1% penicillin/streptomycin, 4 × 10 −4 M monothioglycerol (MTG), 50 μg ml −1 ascorbic acid (Sigma), 200 μg ml −1 transferrin (Boehringer Mannheim) and delivered into the DC-ECM through the connected cannula. To induce CM and SMC specification, RC-DC-ECMs were perfused with basal medium containing human DKK1 (150 ng ml −1 ) and human VEGF (10 ng ml −1 ). To induce more ECs, RC-DC-ECMs were perfused with basal medium containing human VEGF (20 ng ml −1 ) and bFGF (20 ng ml −1 ). Recellularized mouse hearts were perfused using the same growth factor-containing medium for 30 min per time and three times per day (one perfusion every 8 h), and maintained in a 5% CO 2 /5% O 2 /90% N 2 environment. The medium was changed every 48 h. We did not continuously perfuse recellularized hearts as that method washed out most of cells in the first 5 days. Most importantly, we found the periodic perfusion method could consistently make beating heart constructs. In addition, this new method saves time, medium and avoids contaminations during the 14–16 days of perfusion. Cell death and proliferation assessments To detect cell death, terminal deoxynucleotidyl transferase-mediated uridine 5-triphosphatebiotin nick end-labelling (TUNEL) was performed using the In Situ Cell Death Detection Kit, Fluorescein (Roche) according to the manufacturer’s protocol. We used phospho-histone H3 (1:100; Santa Cruz Biotechnology) labelling for cell proliferation assessment. In all, 10 sections/tissue and 3 engineered tissues were calculated. Optical mapping CaiT in the RC-DC-ECM were optically recorded [20] with a high spatiotemporal resolution CMOS camera (Scimedia, Ultima; 1.5 μm × 1.5 μm pixel resolution at 200 frames per second temporal resolution). Briefly, the contracting RC-DC-ECMs was perfused with Tyrode’s solution containing a Ca 2+ indicator (Rhod-2 AM, 10 μg ml −1 , Molecular Probes) at 37 °C for 15 min. A CMOS camera was mounted on an upright microscope (Olympus, BX61WI) to acquire fluorescent images of CaiT. The RC-DC-ECMs were illuminated with a 520±30 nm excitation beam, and the fluorescence from the preparation was collected via a microscope objective lens (× 10 or × 40), passed through a dichroic mirror (565 nm long-pass) and an emission filter (580±30 nm band-pass) and was focused on the CMOS camera to measure CaiT through the Rhod-2 fluorescence. Data analysis was performed using custom-made software [20] . Mechanical testing One end (aorta side) of the engineered tissue was attached to a force transducer (model 401A, Aurora Scientific, Canada) and the other end (ventricular apex side) was connected to a rigid stainless steel wire mounted on a micromanipulator using 10-0 monofilament nylon sutures. The perfusion chamber containing the construct was filled with Tyrode solution (37 °C, 1 ml chamber volume) containing 1.25 mM Ca 2+ . Spontaneous contractions were confirmed by monitoring active force generation using a custom-made analog-digital signal acquisition programme (LabVIEW, National Instruments, Austin, Texas, USA) [28] . The engineered construct was then stimulated using a standard field stimulator (1–2 Hz, 5 ms, 20% above threshold, Harvard Apparatus). We measured: (1) spontaneous contraction force; (2) force–frequency relationship (1–3 Hz frequencies) and (3) response to 5.0 mM external Ca 2+ . Quantitative PCR analysis Real-time quantitative PCR (q-PCR) was performed on a 7900HT Fast Real-Time PCR System (Applied Biosystems) with Fast SYBR Green Master Mix (Applied Biosystems). The results were analysed with EXCEL, normalized to Cyclophilin G ( CYPG ) gene expression, and compared to day 26 EBs. MVP Total RNA from a pool of 10 human fetal hearts was from Agilent Technology. Human atrium total RNA was purchased from Amsbio. Primer sequences are described in Supplementary Table S1 . Statistical analysis All values are reported as mean±s.e.m. of three independent experiments. Statistical analyses were performed by unpaired Student’s t -test. Changes in heart rate following an isoproterenol challenge was run by ANOVA (one-factor repeated ANOVA with post hoc test). A value of P <0.05 was considered significant. How to cite this article: Lu, T.-Y. et al . Repopulation of decellularized mouse heart with human induced pluripotent stem cell-derived cardiovascular progenitor cells. Nat. Commun. 4:2307 doi: 10.1038/ncomms3307 (2013).